Telomeres shorten at equivalent rates in somatic tissues of adults Telomere shortening in somatic tissues largely reflects stem cell replication. Previous human studies of telomere attrition were predominantly conducted on leukocytes. However, findings in leukocytes cannot be generalized to other tissues. Here we measure telomere length in leukocytes, skeletal muscle, skin and subcutaneous fat of 87 adults (aged 19–77 years). Telomeres are longest in muscle and shortest in leukocytes, yet are strongly correlated between tissues. Notably, the rates of telomere shortening are similar in the four tissues. We infer from these findings that differences in telomere length between proliferative (blood and skin) and minimally proliferative tissues (muscle and fat) are established during early life, and that in adulthood, stem cells of the four tissues replicate at a similar rate. Telomere length (TL) is equivalent in different somatic tissues of the human fetus and newborn [1] , [2] , [3] . This equivalence at birth is owing in part to the activity of telomerase [4] , which counteracts TL shortening resulting from cell replication during early intra-uterine growth. During extra-uterine life, telomerase activity is largely repressed in somatic tissues, including in hematopoietic stem cells [5] , [6] ; hence TL varies across somatic tissues in proportion to replicative activity. Notably, leukocyte TL, which reflects TL in hematopoietic stem cells [3] , [7] , is shorter than TLs of minimally proliferative somatic tissues [8] , [9] . Yet, the available data from human studies point to strong correlations in TL across somatic tissues, that is, individuals with long (or short) TL in one tissue also have long (or short) TL in other tissues. This ‘synchrony’ in TL across somatic tissues has been observed not only in humans [1] , [2] , [8] , [9] , [10] but also other mammals, including non-human primates [11] , [12] . Previous reports on the age-dependent attrition of TL in humans are based primarily on studies of leukocytes. These studies suggest that the rate of age-dependent leukocyte TL shortening is rapid early in life but slows down during adulthood in both humans [13] , [14] and in non-human primates [15] . Furthermore, simulations of TL dynamics in granulocytes and leukocytes have been used to gauge the replicative kinetics of hematopoietic stem cells [7] , [16] , [17] . The findings of such simulations suggest that the rapid leukocyte TL attrition during the first two decades of the human life course [7] reflects the expansion of the hematopoietic stem cell and hematopoietic progenitor cell pools. This expansion involves both symmetric cell divisions in which a hematopoietic stem cell divides into two daughter hematopoietic stem cells, and asymmetric cell divisions in which a hematopoietic stem cell divides into one hematopoietic stem cell and one hematopoietic progenitor cell [18] . Growth and development require only a few symmetric replications of hematopoietic stem cells. By contrast, the vast expansion of the hematopoietic progenitor cell pool requires numerous asymmetric replications of hematopoietic stem cells [7] . In this way, the incrementally larger and more differentiated pools and sub-pools of hematopoietic progenitor cells, down the hematopoietic hierarchy, are able to maintain homeostasis of circulating blood cells. During growth and development, homeostasis must accommodate both the expansion of the hematopoietic system and the staggeringly high rate of turnover of some blood cells, which persists throughout life. For instance, ~100 billion neutrophils are mobilized from the bone marrow of adult humans each day [19] . This hierarchical feature of the hematopoietic system explains the infrequent replication of hematopoietic stem cells in adults [7] , [16] , [17] , [20] at the top of the hierarchy in spite of the massive turnover of circulating blood cells at its bottom. It also explains the relatively slow rate of age-dependent leukocyte TL shortening in adulthood [13] , [14] , which largely reflects ‘maintenance’ replicative activity of hematopoietic stem cells, that is, any replicative activity that is not related to growth and development. Data are available about leukocyte TL dynamics (TL and its age-dependent attrition), and by inference these data also enable us to understand much about the replicative kinetics of hematopoietic stem cells in vivo [7] , [16] , [17] , [20] . But no such information exists, to our knowledge, for other somatic tissues. Based on quantifying 14 C in genomic DNA from somatic tissues, skeletal muscle (hereafter referred to as muscle) and fat do experience some replication, presumably of stem cells/progenitor cells [21] , [22] . In the present study, we examined TL measures and age-dependent TL attrition in four tissues in a cross-sectional study spanning more than five decades of adult life. Our findings indicate that during adulthood, age-dependent TL shortening is similar in all four tissues regardless of their replicative activity. This unexpected result provides an important insight with respect to stem cell/progenitor cell replicative kinetics and their potential links to aging and longevity in humans. 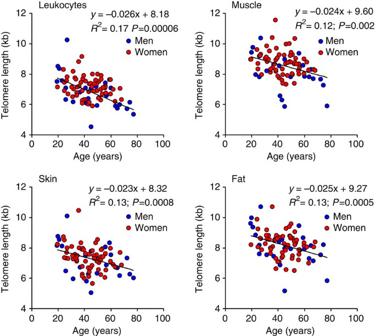Figure 1: Correlation between TL and age in various tissues. TL in leukocytes, muscle, skin and fat is plotted against age. Subject characteristics Participants consisted of 61 women and 26 men ( Table 1 ), 35 Blacks and 52 whites (33 Hispanics and 19 non-Hispanic whites) with an age range of 19–77 years. 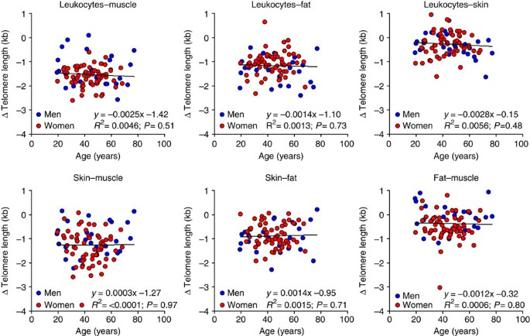Figure 2: Differences in TL in tissues are stable. Differences in TL (Δ) between tissues within the same individuals are plotted against the ages of the donors of the samples. Hispanics and non-Hispanic whites were grouped as whites for comparison with Blacks ( Table 2 ), as no differences were observed between Hispanics and non-Hispanic whites with respect to variables of interest, including TLs in the four tissue types (leukocytes, muscle, skin and fat). Table 1 Demographic characteristics and TL parameters for the entire cohort and by sex. Full size table Table 2 Demographic characteristics and TLs parameters for Blacks and Whites. Full size table TLs of the subjects TL was longest in muscle and shortest in leukocytes ( Table 1 ) ( P <0.0001 (paired Wilcoxon signed-rank test) for all comparisons). In univariate analysis, TL was longer in women than in men for leukocytes and for muscle ( Table 1 ). In addition, Blacks displayed a longer TL than whites in leukocytes and muscle ( Table 2 ). 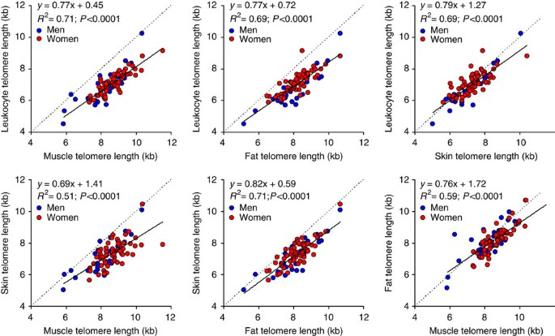Figure 3: Equivalence in TL between tissues within the same individual. Although the correlations between TLs of the four tissues are strong, the highly proliferative tissues (leukocytes and skin) consistently display shorter telomeres than the minimally proliferative tissues (muscle and fat). In multivariable analysis that included age, sex, body mass index and ethnicity/race ( Table 3 ), age explained 17.5% of the inter-individual variation in leukocyte TL, 8.2% of muscle TL, 10.5% of skin TL and 12.4% of fat TL. Table 3 Determinants of tissue TL (univariate and multivariate analysis). Full size table Rates of age-dependent TL attrition Cross-sectional analysis indicated that the four somatic tissues displayed significant but similar age-dependent TL attritions per year (mean±s.e.m. ): leukocytes=26±6 bp; muscle=24±7 bp; skin=23±7 bp; and fat=25±7 bp ( Fig. 1 ). Consequently, the average differences (Δ) in TL between the four tissues were stable throughout the 5-decade age range ( Fig. 2 ). Figure 1: Correlation between TL and age in various tissues. TL in leukocytes, muscle, skin and fat is plotted against age. Full size image Figure 2: Differences in TL in tissues are stable. Differences in TL (Δ) between tissues within the same individuals are plotted against the ages of the donors of the samples. Full size image Comparisons of TLs across somatic tissues TLs in all four tissues displayed wide inter-individual variation in the following ranges: leukocytes=4.52–10.25 kb; muscle=5.86–11.53 kb; skin=5.03–10.44 kb; fat=5.17–10.68 kb ( Table 1 ). Individuals showed strong correlations of TL between tissues, such that those with long (or short) TL in one tissue typically displayed long (or short) TL in other tissues ( r =0.72–0.84, P <0.0001; Pearson’s correlation) for each possible pairing of tissue types ( Fig. 3 ). The association of leukocyte TL with the other three tissues was also consistently high ( r =0.83–0.84, P <0.0001; Pearson’s correlation) for each pairing irrespective of the proliferative nature of the tissue. Figure 3: Equivalence in TL between tissues within the same individual. Although the correlations between TLs of the four tissues are strong, the highly proliferative tissues (leukocytes and skin) consistently display shorter telomeres than the minimally proliferative tissues (muscle and fat). Full size image Three central conclusions can be drawn from this study. First, across more than five decades of adult life, despite different replicative status, leukocytes, muscle, skin and fat displayed similar rates of age-dependent TL attrition. Second, in accord with this result, differences in TLs between the tissues showed no significant change throughout the age range. We infer, therefore, that the TL differences between the tissues were largely established at a younger age, during the first two decades of life. Third, we confirmed observations from previous limited studies that there is an intra-individual synchrony in TL across the somatic tissues of humans [1] , [2] , [3] , [8] , [9] , [10] as evidenced by the strong correlations observed between the TLs in all tissue type pairings. This intra-individual synchrony in TL across somatic tissues is also seen in other mammals [11] , [12] . The finding that four somatic tissues, which are characterized by vastly differing rates of proliferation, showed similar rates of TL attrition across the adult life span was entirely unexpected. A cross-sectional study of ten individuals, including neonates, found no evidence of TL shortening in muscle across more than eight decades [23] . Similarly, another study, comprising 16 subjects (mean age 25 years) and 26 subjects (mean age 74 years), concluded that there was no evidence of age-dependent muscle TL attrition during adulthood [24] . In our much larger, albeit still modestly sized sample population, we used a more accurate method of TL measurement and clearly draw a different conclusion. Longitudinal studies have reported considerable inter-individual variation in the rate of leukocyte TL shortening among adults [25] , [26] . The same presumably applies to TL attrition in other somatic tissues. Although leukocyte TL is largely heritable [27] , [28] , [29] , environmental factors may influence its dynamics. For instance, cigarette smokers [30] , [31] , [32] , obese persons [30] , [31] and those with a sedentary lifestyle [33] , [34] have typically shown shorter leukocyte TLs, presumably owing to an increased burden of inflammation, which might accelerate hematopoietic stem cell divisions, and oxidative stress, which might augment their telomere shortening per replication. Endurance running, in contrast, apparently shortens TL in muscle perhaps owing to heightened proliferation of stem cells/progenitor cells (satellite cells) to build/repair muscle tissue [35] . Thus, the rates of TL attrition in both proliferative and minimally proliferative tissues during adult life may be modified by a variety of factors. This may account in part for the large inter-individual variation of Δ in TLs between tissues within individuals ( Fig. 2 ). Still, as age-dependent TL attrition ultimately reflects division in the stem cell pool, and assuming that telomere loss per division is the same in all somatic tissues, it seems that during adult life the rates of replicative activity of stem cells are similar in proliferative and minimally proliferative tissues. We propose that the differences in TL between somatic tissues of adults largely arise from the expansion during growth and development of the stem cell pool through both symmetric stem cell divisions and more so for the progenitor cell pool, through asymmetric stem cell divisions. Theoretically, <5 rounds of symmetric divisions of the entire hematopoietic stem cell pool are necessary to expand the compartment in tandem with an increase in body weight from 3 kg of birth weight to 80 kg adult weight, that is, 3–6 kg (first round); 6–12 kg (second round); 12–24 kg (third round); 24–48 kg (fourth round); and 48–96 kg (fifth round) [7] . Therefore, to accommodate growth, the impact of the expansion of the hematopoietic stem cell pool on leukocyte TL is relatively small. This is also likely to be the case for TL dynamics in other somatic tissues, including minimally proliferative ones. In contrast, numerous asymmetric divisions of hematopoietic stem cells are required during growth to build the large hematopoietic progenitor cell pool in order to maintain the numbers of circulating blood cells, a subset of which has an enormous turnover [19] . Consequently, as illustrated in Fig. 4 , leukocyte TL undergoes considerable shortening during early life [7] , [13] , [14] , [15] . The same might apply, although to a lesser extent, to other highly replicative somatic tissues, such as skin. In contrast, the expansions of progenitor cell pools during growth and development in minimally proliferative tissues, such as muscle and fat, are probably limited. The sizes of these progenitor cell pools may be calibrated to accommodate only small cell turnover rates in adulthood. Accordingly, early in life, TLs of muscle and other minimally proliferative tissues undergo substantially less attrition than leukocyte TL ( Fig. 4 ). The need to establish a huge hematopoietic progenitor cell pool may be the reason that bone marrow failure is the first catastrophic manifestation arising from major mutations in telomere maintenance genes [36] . It also explains the rapid leukocyte TL shortening post hematopoietic stem cell transplant [37] , with the rebuilding of both the hematopoietic stem cell pool and also the hematopoietic progenitor cell pool. Nevertheless, the strong correlations noted between all pairings of tissue types, irrespective of their replicative potential, suggest that the initial equivalence of TL in utero and at birth [1] , [2] continues to dominate the TL phenotypic landscape across the lifespan, and that accelerated stem cell division during growth and development after birth exerts a more modest effect that reduces this equivalence. Thus, the main contributors to TL and its similarity in individuals are primarily prenatal, followed by growth in childhood and adolescence, with less influence in adulthood. 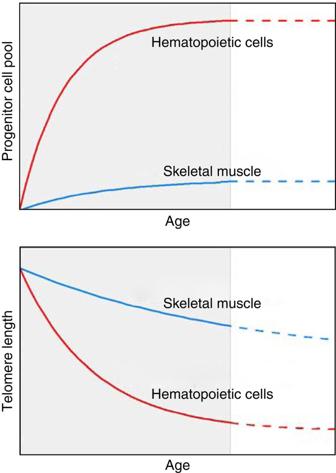Figure 4: Model of progenitor cell pool dynamics and in different tissues. Upper panel: during growth (grey shade), the progenitor cell pool in the hematopoietic system undergoes massive expansion through asymmetric replication of hematopoietic stem cells. In this way, the system can accommodate the tremendous turnover in peripheral blood cells. In contrast, during growth, the progenitor cell pool in skeletal muscle undergoes a modest expansion through replication of muscle stem cells, as the turnover of skeletal muscle cells is small. Lower panel: reflecting the expansions of the progenitor cell pools in the respective systems, TL undergoes rapid attrition in the hematopoietic system but only modest attrition in skeletal muscle. The slow and parallel attritions of TLs in stem cells, as expressed in leukocyte TL and in skeletal muscle TL during adult life, are the outcome of ’maintenance’ replicative activities of stem cells/progenitor cells in these systems. Figure 4: Model of progenitor cell pool dynamics and in different tissues. Upper panel: during growth (grey shade), the progenitor cell pool in the hematopoietic system undergoes massive expansion through asymmetric replication of hematopoietic stem cells. In this way, the system can accommodate the tremendous turnover in peripheral blood cells. In contrast, during growth, the progenitor cell pool in skeletal muscle undergoes a modest expansion through replication of muscle stem cells, as the turnover of skeletal muscle cells is small. Lower panel: reflecting the expansions of the progenitor cell pools in the respective systems, TL undergoes rapid attrition in the hematopoietic system but only modest attrition in skeletal muscle. The slow and parallel attritions of TLs in stem cells, as expressed in leukocyte TL and in skeletal muscle TL during adult life, are the outcome of ’maintenance’ replicative activities of stem cells/progenitor cells in these systems. Full size image We acknowledge a number of shortcomings of this study. First, our study was cross-sectional in design; we used tissues obtained during elective surgical procedures from individuals of different ages to compute TL dynamics. Ideally, measurement of age-dependent TL attrition should be performed longitudinally in the same individuals, but this was simply not feasible. Second, the samples of muscle, skin and fat were obtained from different sites, but we doubt that body region exerted any influence on the findings. We found no evidence that surgical site (head and neck, thorax, abdomen, upper extremities and lower extremities) impacted TL without and with adjustment for age. Third, leukocyte TL is derived from circulating cells, which are partitioned from the less mature hematopoietic cells in the bone marrow. In contrast, TLs in solid tissues reflect TL of fully differentiated cells as well as resident stem cells/progenitor cells. However, we doubt that TLs of these precursor cells exert an appreciable influence on the mean TLs in muscle and other minimally proliferative tissues, because, as discussed above, the size of the stem cell/progenitor cell pools in these tissues is very small. Furthermore, although we examined several fold more patients than in previous studies, our sample size remains modest and requires extension. In conclusion, in adults, both highly proliferative and minimally proliferative tissues appear to display similar age-dependent telomere attrition. Moreover, in this study population, the average gap in TLs between the proliferative and minimally proliferative tissues was essentially constant between the ages of 19–77 years, suggesting that the first 20 years of life is a crucial time period for establishing this difference. As TL dynamics largely reflect stem cell kinetics, we infer that stem cell division rates for maintenance might be similar in the somatic tissues we examined, regardless of their proliferative status. Making clinical use of TL in predicting future health risks will depend to a large extent on understanding the underlying inter-individual variations in TL at birth and its attrition during human growth and development. Recruitment of study participants Inpatients and outpatients scheduled for general, plastic and vascular surgery at the University Hospital of the University of Medicine and Dentistry of New Jersey were approached by the study coordinator for participation in this investigation. These also included patients undergoing surgical procedures to remove cancer with no evidence of metastasis. This research was approved by the Institutional Review Board (IRB) of the University of Medicine and Dentistry of New Jersey, New Jersey Medical School. All participants signed a written informed consent approved by the IRB. Participants were asked to donate blood (from the intravenous line or phlebotomy) and ~50–100 mg specimens of skin, subcutaneous fat and skeletal muscle in the surgical field. If the attending surgeon indicated the study coordinator that one of the tissue types could not be sampled during the surgery, the potential study subject was not approached for enrolment. Similarly, all subjects who had received therapeutic irradiation to the surgical site and those with a history of immunosuppression secondary to a medical condition or of chemotherapy for cancer treatment were not enroled. Three subjects were excluded owing to HIV infection and sickle cell disease. Measurements of TL DNA integrity was evaluated by resolving samples on 1% (wt/vol) agarose gel. Samples were digested with restriction enzymes Hinf I (10 U) and Rsa I (10 U; Roche). Digested DNA samples and DNA ladders were resolved on 0.5% agarose gels. After 16 h, the DNA was depurinated for 15 min in 0.25 N HCl, denatured 30 min in 0.5 M NaOH/1.5 mol l −1 NaCl and neutralized for 30 min in 0.5 mol l −1 Tris, pH 8/1.5 M NaCl. The DNA was transferred for 1 h to a positively charged nylon membrane (Roche) using a vacuum blotter (Boeckel Scientific, Feasterville, PA). Membranes were hybridized at 65 o C with the DIG-labelled telomeric probe overnight as previously described [38] . The DIG-labelled probe was detected by the DIG luminescent (Roche) and exposed on X-ray film. The inter-assay coefficient of variation of the TL measurements was 1.8%. Statistical analysis Descriptive values are expressed as mean±s.d., number of patients and percentages. The population was divided according to sex or ethnicity/race, and compared using the Wilcoxon rank-sum test or the χ 2 test. Comparisons of TL among different tissues were performed using a paired Wilcoxon signed-rank test. A P -value <0.05 was regarded as statistically significant. Relationships between TL and age in the four tissues (by pairs) were determined using Pearson’s correlation coefficients. The effects of age, sex, race/ethnicity and body mass index were evaluated in a multiple regression analysis by including the variables associated with TL that had a P -value <0.10 in the univariate analysis. Statistical analyses were carried out using the NCSS 2004 statistical software package. How to cite this article: Danial, L. et al . Telomeres shorten at equivalent rates in somatic tissues of adults. Nat. Commun. 4:1597 doi: 10.1038/ncomms2602 (2013).